Methylotrophic methanogenic Thermoplasmata implicated in reduced methane emissions from bovine rumen Rumen methanogens are major sources of anthropogenic methane emissions, and these archaea are targets in strategies aimed at reducing methane emissions. Here we show that the poorly characterised Thermoplasmata archaea in bovine rumen are methylotrophic methanogens and that they are reduced upon dietary supplementation with rapeseed oil in lactating cows. In a metatranscriptomic survey, Thermoplasmata 16S rRNA and methyl-coenzyme M reductase ( mcr ) transcripts decreased concomitantly with mRNAs of enzymes involved in methanogenesis from methylamines that were among the most abundant archaeal transcripts, indicating that these Thermoplasmata degrade methylamines. Their methylotrophic methanogenic lifestyle was corroborated by in vitro incubations, showing enhanced growth of these organisms upon methylamine supplementation paralleled by elevated methane production. The Thermoplasmata have a high potential as target in future strategies to mitigate methane emissions from ruminant livestock. Our findings and the findings of others also indicate a wider distribution of methanogens than previously anticipated. Ruminant livestock is a major global source of methane (CH 4 ) [1] , [2] . The digestive fermentation activity of ruminants accounts for ~37% of anthropogenic CH 4 emissions [2] . CH 4 is the end product of a complex anaerobic degradation pathway of plant biomass by the ruminal microbiota, the terminal group being methanogenic archaea. H 2 is the major energy source of rumen methanogens known to date [3] , and these archaea are targets in strategies aimed at reducing CH 4 emissions. With global demands for milk and meat expected to double by 2050, CH 4 emissions are predicted to increase accordingly [4] . Ruminal CH 4 production also represents an energy loss to the animal [5] ; hence, reducing methanogenesis is of both environmental and economic interest. Until recently, rumen methanogens have been found to belong to a few genera of the Methanobacteriales and Methanomicrobiales orders within the phylum Euryarchaeota [3] . These orders have all been characterised as hydrogenotrophic, utilizing H 2 /CO 2 or H 2 /methanol produced by various fermentative bacteria in the process of anaerobic degradation of plant biomass. A novel group [6] distantly related to the Thermoplasmatales (recently named ‘rumen cluster C’ (RCC) [3] ; previously described as rice cluster C Thermoplasmata [7] ) was found to be highly abundant in ruminants based on 16S ribosomal RNA (rRNA) genes [3] . No representatives of the RCC Thermoplasmata have been isolated, although their methanogenic lifestyle was proposed because of the parallel presence of distinct methyl-coenzyme M reductase genes ( mcr ) [3] , [8] , [9] . However, the recently described Methanomassiliicoccus luminyensis isolated from human feces from the related rice cluster III clade provided evidence for methanogenic Thermoplasmata [10] . Approaches to reduce CH 4 emission from livestock, such as dietary supplementation of unsaturated fatty acids [11] , typically focus on reducing H 2 availability for rumen methanogens. However, because of the complexity of the rumen microbiota, results are not fully predictable and the effects of the manipulations are poorly understood [12] . Here, for the first time, a metatranscriptomic approach was used to investigate the in vivo effect of rapeseed oil (RSO) supplementation on the rumen microbiota of lactating Holstein cows, with particular focus on methanogenic archaea. We show that the poorly characterised Thermoplasmata in bovine rumen are a novel group of methylotrophic methanogens and that they are reduced upon CH 4 mitigation in lactating cows. Effect of RSO supplementation on CH 4 emission RSO supplementation significantly reduced CH 4 emission, as shown by a 6.2% lower CH 4 -to-CO 2 emission ratio ( P <0.05; Supplementary Table S1 ). In a previous experiment with identical diets, CH 4 -to-CO 2 ratio was reduced by 8.5% upon RSO supplementation, corresponding to an 18% reduction in emitted CH 4 per energy corrected milk yield [13] ( Supplementary Table S1 ). Rumen metatranscriptomics A metatranscriptomics approach with random-hexamer primed reverse transcription was applied on rumen fluid to simultaneously assess the impact of RSO on the abundance of rumen microorganisms and their gene expression [14] (see Methods). Illumina deep-sequencing with overlapping read paired-end technology [15] resulted in ~10–12 million high-quality reads of ~160-bp length per sample. Although the majority of sequences represented rRNA (‘ribo-tags’), between 380,000 and 485,000 sequences were putative messenger RNAs (mRNAs) ( Supplementary Table S2 ). A three-domain profile of the rumen microbiota revealed that Bacteria and Eukaryotes each contributed approximately 50% of ribo-tags, whereas Archaea were present at approximately 1% ( Supplementary Fig. S1 ; see Supplementary Figs. S2 and S3 for a complete overview of bacterial and eukaryotic communities, respectively). The Archaea was constituted by Methanobacteriales (genera Methanobrevibacter and Methanosphaera ) and the RCC Thermoplasmata. Surprisingly, only the RCC decreased significantly ( P <0.05) with RSO supplementation ( Fig. 1 ), indicating that they were associated with the reduction in CH 4 , whereas the well-studied Methanobacteriales were not. Likewise, the mRNA levels of the key-enzyme methyl-coenzyme M reductase (Mcr) were reduced upon RSO amendment ( Fig. 1 ). Remarkably, transcripts of all three subunits α, β and γ of Mcr were affected ( Fig. 1 ). The decrease of mcrA transcripts was corroborated by quantitative PCR (qPCR) ( Supplementary Table 3 ). 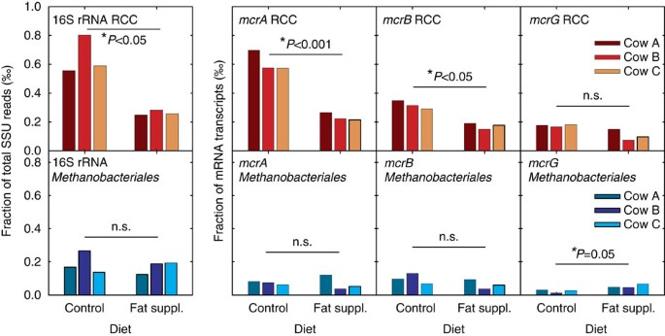Figure 1: Effect of RSO on methanogensin vivo. Relative abundances of transcripts from RCC (upper row) and fromMethanobacteriales(bottom row) from individual cows on control and rapeseed oil (RSO)-supplemented diets, respectively. Relative fraction of archaeal SSU ribo-tags affiliated to RCC andMethanobacterialesis shown as % of total SSU reads, and fraction ofmcrA,mcrBandmcrGtranscripts detected for RCC and other methanogens (that is,Methanobrevibacter ruminantiumandMethanosphaera stadtmanae), shown as ‰ of all mRNA transcripts with a significant homologue in Genbank nr (e-value<1e-5) for each sample.P-values ≤0.05 are considered representing significant effects of fat supplementation (*marked) using pairedt-test. ThemcrGof RCC was trend-wise affected by fat supplementation (P<0.10). n.s., not significant; suppl, supplement. 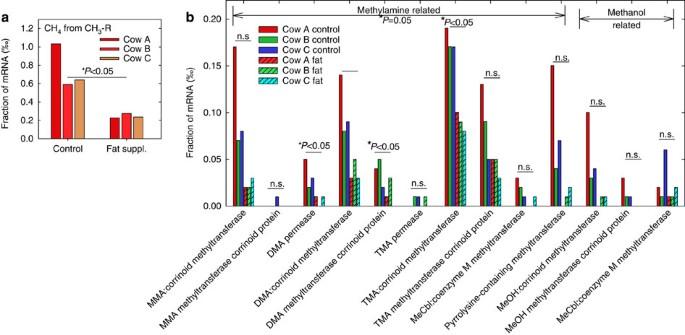Figure 3: Transcripts of methanogenesis from methylamines. Effect of RSO amendment on the expression of SEED functional gene categories of (a) methanogenesis from methylated compounds combined and (b) transcripts for utilizing MAs and methanol as substrates for CH4production inferred from a global functional analysis of all mRNAs with MEGAN using the SEED functional categories. MMA, monomethylamine; DMA, dimethylamine; TMA, trimethylamine; MeCbl, methylcobalamine; MeOH, methanol.P-values ≤0.05 are considered representing significant effects of fat supplementation (*marked) using pairedt-test. n.s., not significant; suppl, supplement. Figure 1: Effect of RSO on methanogens in vivo . Relative abundances of transcripts from RCC (upper row) and from Methanobacteriales (bottom row) from individual cows on control and rapeseed oil (RSO)-supplemented diets, respectively. Relative fraction of archaeal SSU ribo-tags affiliated to RCC and Methanobacteriales is shown as % of total SSU reads, and fraction of mcrA , mcrB and mcrG transcripts detected for RCC and other methanogens (that is, Methanobrevibacter ruminantium and Methanosphaera stadtmanae ), shown as ‰ of all mRNA transcripts with a significant homologue in Genbank nr ( e -value<1 e -5) for each sample. P -values ≤0.05 are considered representing significant effects of fat supplementation (*marked) using paired t -test. The mcrG of RCC was trend-wise affected by fat supplementation ( P <0.10). n.s., not significant; suppl, supplement. Full size image Mcr transcript assembly using the CAP3 program resulted in full-length sequences of the three mcr subunits α, β and γ, among shorter contigs. Although several of the short contigs were highly similar to mcr subunits of Methanobrevibacter and Methanosphaera , the long contigs were only distantly related to mcr of Methanobrevibacter and Methanosphaera or to other cultured methanogens (<70% DNA similarity) ( Fig. 2a ). However, mcrA was >95% similar to partial mcrA genes associated with the RCC archaea (for example Evans et al. [9] and Acc. nos. JN229252/JN229233). Based on this, all three subunits were assigned to RCC. We validated this approach through assembly of the archaeal transcripts of elongation factor 1α (EF-1α) and 16S rRNA. Phylogenetic reconstruction of a translated amino-acid sequence of the obtained full-length EF-1α revealed an association with EF-1α of the Thermoplasmata branch of Euryarchaota ( Fig. 2b ), which is similar to the placement of the 16S rRNA of RCC ( Fig. 2c ). Assignment of all single mcr transcripts to the full-length mcr genes of the RCC clade and the Methanobacteriales revealed a significant decrease of mcrA and mcrB transcripts of RCC upon RSO amendment ( P <0.05; Fig. 1 ), and not of the Methanobacteriales . 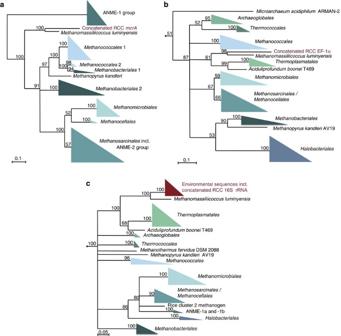Taken together with the 16S rRNA data, this gives evidence that the RCCs were responsible for the decreased CH 4 emissions. Figure 2: Phylogenetic analysis of RCC Thermoplamata. Maximum likelihood phylogenetic analyses of concatenatedmcrA, EF-1α and 16S rRNA sequences of RCC. (a) McrA phylogeny based on an amino-acid alignment (569 positions after removal of ambigiously aligned sites and 100 bootstraps). The scale bar refers to 10% estimated sequence divergence. (b) EF-1α phylogeny based amino-acid alignment (368 positions) (removal of ambiguously aligned sites, 50% indel filter and 100 bootstraps). The tree was rooted with corresponding sequences from Cren-, Kor- and Thaumarchaeota. The scale bar refers to 10% estimated sequence divergence. (c) 16S rRNA phylogeny based on nucleotid alignment (1212 positions) (removal of ambigiously aligned sites and 100 bootstraps). Thaumarchaeal 16S rRNA sequences were used as outgroup. The scale bar refers to 5% sequence divergence. Nodes with bootstrap value >50 were kept, whereas those <50 were removed and are shown as multifurcations. Figure 2: Phylogenetic analysis of RCC Thermoplamata. Maximum likelihood phylogenetic analyses of concatenated mcrA , EF-1α and 16S rRNA sequences of RCC. ( a ) McrA phylogeny based on an amino-acid alignment (569 positions after removal of ambigiously aligned sites and 100 bootstraps). The scale bar refers to 10% estimated sequence divergence. ( b ) EF-1α phylogeny based amino-acid alignment (368 positions) (removal of ambiguously aligned sites, 50% indel filter and 100 bootstraps). The tree was rooted with corresponding sequences from Cren-, Kor- and Thaumarchaeota. The scale bar refers to 10% estimated sequence divergence. ( c ) 16S rRNA phylogeny based on nucleotid alignment (1212 positions) (removal of ambigiously aligned sites and 100 bootstraps). Thaumarchaeal 16S rRNA sequences were used as outgroup. The scale bar refers to 5% sequence divergence. Nodes with bootstrap value >50 were kept, whereas those <50 were removed and are shown as multifurcations. Full size image Methylotrophic methanogenesis from methylamines (MAs) Although the RCC clade has been previously suggested as a novel order of methanogens [3] , [8] , [9] , information on the pathway of methanogenesis was not available. A global functional analysis of all mRNAs with MEGAN using the SEED functional categories [16] revealed the presence of transcripts for the methanogenic pathways with methylated compounds as substrates ( Fig. 3a ). These were similar in abundance to transcripts of the ‘core methanogenesis’, and likewise decreased significantly upon RSO treatment ( P <0.05, Supplementary Fig. S4a ). Closer inspection identified transcripts for utilization of tri-, di- and monomethylamine and methanol, pointing to these substances as important substrates for the rumen methanogens ( Fig. 3b ). Especially, the presence of transcripts for utilization of MAs is remarkable, because Methanosarcinaceae were until now the only methanogens known to grow on these substrates. Furthermore, all enzymes in the three MA pathways were only distantly related to those from Methanosarcinaceae (<66% amino-acid sequence identity, Supplementary Table S4 ). The first enzymes in these pathways are corrinoid-dependent MA methyltransferases (Mt1 [17] ); these contain the unique, reactive amino-acid pyrrolysine (the 22 nd aa), encoded via an in-frame stop codon on the mRNA, as a conserved trait [17] . All putative mt1 transcripts harboured this stop codon, making it highly likely that these indeed encode functional Mt1 enzymes. In summary, the metatranscriptomic data strongly suggest that RCCs are a novel order of methylotrophic methanogens, obtaining energy and carbon from MAs derived from the degradation of betaine and choline, and possibly also from methanol. Additional evidence for this methylotrophic methanogenic lifestyle comes from the recently isolated Methanomassiliicoccus luminyensis of the closely related rice cluster III, which was isolated with H 2 /methanol as substrate. A screening of the M. luminyensis genome [18] with the RCC transcripts revealed the presence of all genes for methanogenesis from MA ( Supplementary Table S4 ). Also very recently, a methanogenic enrichment from the termite gut was dominated by Thermoplasmata utilizing H 2 /methanol [19] . Figure 3: Transcripts of methanogenesis from methylamines. Effect of RSO amendment on the expression of SEED functional gene categories of ( a ) methanogenesis from methylated compounds combined and ( b ) transcripts for utilizing MAs and methanol as substrates for CH 4 production inferred from a global functional analysis of all mRNAs with MEGAN using the SEED functional categories. MMA, monomethylamine; DMA, dimethylamine; TMA, trimethylamine; MeCbl, methylcobalamine; MeOH, methanol. P -values ≤0.05 are considered representing significant effects of fat supplementation (*marked) using paired t -test. n.s., not significant; suppl, supplement. Full size image Methylotrophic methanogenesis from MA was verified in vitro by adding trimethylamine (TMA) to bovine rumen fluids. Incubation with 15 mM TMA resulted in a 22% increase ( P <0.01) of CH 4 in the headspace by 24 h ( Fig. 4a ), whereas the addition of the methanogenesis inhibitor bromoethanesulfonic acid completely inhibited CH 4 formation ( Supplementary Fig. S5 ). This confirmed the ability of rumen methanogens to quickly utilize TMA. Abundance of RCC methanogens, as determined by qPCR of 16S rRNA and TMA methyltransferase ( mttB) genes, increased threefold in the presence of TMA. In contrast, growth of other methanogens was independent of TMA addition as indicated by comparable increase of 16S rRNA gene copies in both control and TMA supplemented samples, respectively ( Fig. 4b and Supplementary Fig. S6 ). 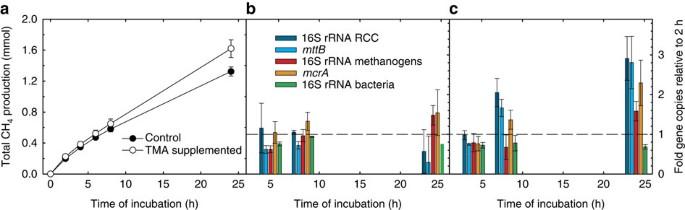Figure 4: Methanogenesis from TMA by RCCin vitro. CH4production (a) without and with TMA (15 mM), and concurrent x-fold change in bacterial, methanogen and RCC 16S rRNA genes,mttBandmcrAin rumen fluid fermentations (b) without and (c) with TMA, as quantified by qPCR. X-fold change in gene copies was calculated relative to 2 h. Total CH4production differed significantly between treatments after 24 h (non-pairedt-test;P<0.01). Error bars represent s.d. of quadruple incubations. TMA, trimethylamine;mttB, TMA methyltransferase;mcrA, methyl-coenzyme M reductase subunit α. Figure 4: Methanogenesis from TMA by RCC in vitro . CH 4 production ( a ) without and with TMA (15 mM), and concurrent x-fold change in bacterial, methanogen and RCC 16S rRNA genes, mttB and mcrA in rumen fluid fermentations ( b ) without and ( c ) with TMA, as quantified by qPCR. X-fold change in gene copies was calculated relative to 2 h. Total CH 4 production differed significantly between treatments after 24 h (non-paired t -test; P <0.01). Error bars represent s.d. of quadruple incubations. TMA, trimethylamine; mttB , TMA methyltransferase; mcrA , methyl-coenzyme M reductase subunit α. Full size image Sources of MAs and rumen nitrogen cycling Formation of TMA from glycine betaine and (phosphatidyl-) choline by rumen bacteria and of CH 4 from MAs has been shown during the last decades [20] , [21] , [22] , [23] . The identification of methylotrophic RCC finally identifies the responsible methanogens. Especially, glycine betaine is present in high amounts in feeds containing beet pulp, which was also included in the diet used in this study (see Supplementary Table S5 for details). This might also explain the comparably high abundance of RCC compared with other studies [3] . As the degradation of MAs leads to the release of ammonium (NH 4 + ) [20] , [21] , the utilization of MAs by RCC has implications for the entire rumen bacterial community. Intriguingly, the metatranscriptomic data also revealed a decrease of 30–60% of transcripts for NH 4 + assimilation in the RSO-supplemented cows ( Supplementary Fig. S4b ), suggesting that RCC constitute an additional supplier of NH 4 + in the rumen, besides NH 4 + derived from protein degradation. Inhibitory effect of RSO In order to obtain an estimate about the concentration of MAs in the rumen fluids and to obtain insights into the inhibitory effect of RSO on RCC, we quantified TMA using direct infusion Orbitrap mass spectrometry (see Methods). The TMA concentrations were approximately 40 μM in the controls and increased about fivefold to 220 μM in RSO samples. These data show that (1) substantial amounts of TMA were present in the rumen fluids and (2) that TMA did not become limiting in the RSO samples. The latter indicates that the inhibitory effect of RSO on RCC is not via substrate limitation. Rather, RSO components (for example, glycosinolates) might have been directly or indirectly toxic for RCC. This conclusion is supported by the fact that no consistent change in the rumen bacterial community composition of replicate samples was observed with RSO amendment ( Supplementary Fig. S2 ), as it would have been expected in the case of indirect RSO effect via shifts in the metabolic pathways, leading to substrate limitations for RCC. This study provides compelling evidence that the RCC clade of Thermoplasmata is a novel group of methylotrophic methanogens in the bovine rumen with MAs as their major energy and carbon sources. It is currently unclear whether RCC are also hydrogenotrophic or not, however, our data show that RCC occupy a niche separate from the other rumen methanogens. Nevertheless, this study showed that RCC, rather than solely hydrogenotrophic methanogens, are the primary target of CH 4 mitigation via RSO supplementation. Because the RCC clade has been detected in many ruminants worldwide [3] , our findings suggest new possibilities for CH 4 mitigation strategies for dairy cows, either by targeting the RCC directly or via dietary supplements focusing on MA, and not on H 2 , for mitigating ruminal CH 4 production. Still, long-term feeding experiments are needed to uncover the true potential of RCC as targets for CH 4 mitigation strategies. The identification of methanogenic organisms in the Thermoplasmata branch of the archaeal phylum Euryarchaeota in this study and other studies [10] , [19] published during the review process of this work substantiates previous theories about the widespread occurrence of this potentially primordial metabolism that probably developed early in evolution and was in the common ancestor of all Euryarchaeota [24] , perhaps even of all archaea. It is also noteworthy that this branch of Thermoplasmata harbours several other groups devoid of cultivated representatives, which have been detected in rice field soils, marine sediments and other presumably anoxic habitats [7] , indicating a previously unrecognized, wider ecological distribution of methanogenic archaea [19] . Diets and experimental setup Four Holstein dairy cows were fed two different diets, a control (total fat content of 3.5% of dry matter (DM)) and a RSO-supplemented diet (supplemented with 33 g RSO per kg feed, resulting in a total fat content of 6.5% of DM; Supplementary Table S5 ), in a conventional 4 × 2 cross-over design where two cows were fed the low fat-control diet and two cows were fed the fat-supplemented diet during the first period, and vice versa during second period. Each feeding period lasted for 3 weeks and the cows were fed twice daily during the entire period. The animal experiment was designed and approved by The Experimental Animal Inspectorate under The Danish Ministry of Justice (2008/561–1500), and completed with the highest consideration for the well being of the cows. However, one cow was excluded from the full experiment because of health considerations, which were not related to the feed manipulation. Quantification of CH 4 emission from dairy cows CH 4 emission from the cows was quantified using custom-built transparent polycarbonate chambers (1.83 × 3.82 × 2.45 m) located in the barn. The cows were housed individually, and quantification of CH 4 and CO 2 emission from each cow was performed over two times 48 h during the last week of each feeding period. The air flow through the chambers was measured with a mass flow meter (Teledyne Hastings Instruments, Hampton, VA, USA), and CO 2 and CH 4 was quantified using infrared sensors (Columbus Instruments, Columbus, OH, USA) exactly as described in Hellwing et al. [25] Nucleic acid extraction and double-stranded (ds) cDNA synthesis Rumen fluid-sampling strategy was developed from previous publications [26] , [27] , [28] , taking into account that a significant fraction of the rumen microbiota is adhered to fibers. Hence, representative samples of rumen fluid were collected at the end of each feeding period from the top and bottom part of the frontal, mid and distal section of the rumen (25 ml from each area) through a rumen fistula. The rumen fluid was pooled in sterile plastic bags with filter inserts (pore size 0.5 mm, Grade Blender Bags; VWR - Bie & Berntsen, Denmark), physically disrupted to release microorganisms from fibers into the rumen fluid, enabling sampling of rumen fluid representing both the fiber-adhered and the always occurring rumen fluid community. Finally, rumen fluid was sieved and decanted into 1.5 ml Eppendorf tubes, snap frozen in liquid nitrogen and stored at −80 °C until nucleic acid (NA) extraction. NAs were extracted using a standard phenol-chloroform bead-beating procedure. RNA was further purified using the NucleoSpin RNA Clean-up XS (Macherey-Nagel). RiboLock RNase inhibitor was added to purified RNA samples. The contaminated DNA was removed from the combined RNA/DNA extracts through the use of the DNase I kit (Fermentas). The absence of DNA was verified by PCR targeting the 16S rRNA gene ( Supplementary Table S6 ). DNase -treated RNA was purified using the MEGAclear kit (Invitrogen). Total RNA was quantified using a NanoDrop-1000 (Thermo Fisher Scientific, Waltham, MA, USA) and quality of the purified RNA was tested using the Experion RNA StdSens Analysis Kit (BioRad, Hercules, CA, USA). The synthesis of double-stranded cDNA was performed using the SuperScript Double-Stranded cDNA Synthesis Kit (Invitrogen) as previously described [29] . Sequencing and bioinformatic analysis Sequencing of the samples was performed on the Illumina HiSeq2000 system (BGI, Shenzhen, Hong Kong) using fragmented ds cDNA (≈160 bp; paired-end sequenced from 2 × 100 bp read lengths). Paired-end reads were assembled using the SHE-RA software [15] . Concatenated sequences were filtered using a 60% quality confidence cutoff. Small subunit (SSU) rRNAs were analysed according to Urich et al. [14] ; putative mRNA-related reads were analysed using Meta-Genome Rapid Annotation using Subsystems Technology, v. 3.1.2. ( http://metagenomics.anl.gov/ ) with subsystem-based annotation based on the SEED database [30] and with MEGAN4 [31] analysis of BlastX searches against the Genbank Refseq protein database (with e -value cutoff 1 e −5 ). Mcr transcripts were identified with BlastN searches against the data sets (with e -value cutoff 1 e −5 ) using representative gene sequences. Assembly of transcripts was done with CAP3 (ref. 32 ). Elongation factor 1α and mcrB transcripts were assembled with stringent parameters –p90 –o50; mcrA and mcrG were assembled with –p95 –o50. Taxonomically, pre-binned RCC 16S ribo-tags were assembled with default parameters. McrA, EF-1α and 16S rRNA phylogeny reconstruction Sequences were downloaded from NCBI and the Functional Gene Pipeline/Repository homepage ( http://fungene.cme.msu.edu/ ). McrA and EF-1α protein sequences, as well as 16S rRNA genes, were aligned using clustalW2 (ref. 33 ) from European Bioinformatics Institute (EBI). Alignments were manually corrected in BioEdit [34] , and ambiguously aligned positions were removed (a 50% indel filter was applied for the EF-1α alignment). Phylogenetic analyses were performed with the Maximum Likelihood (PhyML) software [35] using default parameters and 100 bootstraps, and phylogenies were visualized with NJPlot [36] . Quantification of mcrA gene copies by qPCR Quantification of methanogen mcrA gene copies in ds cDNA was done using the Roche Lightcycler 480 instrument (Roche, Mannheim, Germany). Each reaction (20 μl) consisted of 10 μl of Sybr Green I Master Mix (Roche), 1 μl each of mlas for forward primer and mcrA-rev reverse primer (10 pmol μl −1 ) ( Supplementary Table S6 ), 7 μl of ddH 2 O and 1 μl of ds cDNA template at a concentration of approximately 10 ng μl −1 (ds cDNA concentration quantified using NanoDrop-1000, Thermo Fisher Scientific). Running conditions were 95 °C for 3.5 min followed by 40 cycles of 92 °C for 30 s, 55 °C for 45 s and 72 °C for 30 s. Acquisition of fluorescent signal was done at 83 °C (15 s) after each cycle. Product specificity and size was confirmed by melting point analysis and by agarose gel electrophoresis, respectively. Detection range for mcrA gene copies was between 10 1 and 10 9 gene copies per μl in the standards prepared for qPCR (slope: −3.362, efficiency: 1.983, error: 0.0124). Rumen fluid incubations with TMA Rumen fluid was sampled from a rumen fistulated Holstein breed dairy cow fed a maintenance diet [37] . Rumen fluid was sampled before morning feeding from the top and bottom part of the frontal, mid and distal section of the rumen (300–400 ml rumen fluid from each site), mixed and sieved through a sterile filter bag with a pore size of 0.5 mm (VWR) into a sterile 2-l blue-cap bottle flushed with an anoxic nitrogen gas. Rumen fluid (50 ml) was poured into each of eight sterile N 2 gas flushed infusion bottles with 10 ml 0.1 M sodium phosphate buffer (anaerobic, pH 6.5). All bottles were sealed using gas-impermeable rubber stoppers and acclimated in a thermo-controlled shake incubator (38 °C, 30 min, 80 r.p.m.). Right at the beginning of the experiment, the bottles were flushed with a gas mix consisting of 10% H 2 , 10% CO 2 and 80% N 2 ; TMA (Sigma-Aldrich, St. Louis, MO, USA) was added to four bottles (15 mM, final concentration). All bottles were again incubated (38 °C, 80 r.p.m.). Gas samples were taken at 0, 2, 4, 6, 8 and 24 h and immediately analysed by gas chromatography using a ML GC82-22 (Mikrolab, Aarhus, Denmark) with helium as carrier gas. Data were analysed using the appurtenant PEAK359 software. N 2 gas in the bottles was used as internal standard for calculating H 2 , CO 2 and CH 4 production in the rumen fluid. Rumen fluid was sampled simultaneously with gas samples, snap frozen in liquid nitrogen and stored at −80 °C. The pH was measured in all bottles after 24 h. An additional 6-h in vitro incubation experiment was performed with six bottles, with rumen fluid and buffer as described above, under a 100% N 2 atmosphere. Two bottles were supplemented with TMA (10 mM), two bottles with TMA and bromoethanesulfonic acid (20 mM), and two bottles represented control treatments. Gas samples were taken after 0, 1, 2, 3, 4 and 6 h and analysed as described above. Quantification of TMA in rumen samples using direct infusion Orbitrap mass spectrometer A volume of 1 ml rumen fluid from each cow at each diet was centrifuged in Eppendorf tubes for 15 min at 20 000 r.p.m. at 4 °C. Approximately 800 μl supernatant was transferred to new Eppendorf tubes and frozen at −20 °C. In all, 50 μl of sample was diluted with an equal amount of buffer solution (MeOH:H 2 O=50:50, 0.1% formic acid) containing 0.1 mg ml −1 15N-labeled internal standard (TMA*HCl, Sigma-Aldrich). Samples were analysed with a LTQ-Orbitrap XL mass spectrometer equipped with a nano electrospray ion source (Thermo Fisher Scientific, Bremen, Germany) using direct infusion at a flow rate of 1 μl min −1 . Spectra were recorded with the high-resolution Fourier-Transformation mass analyzer. The system was rinsed between sample injections with buffer solution for at least 20 min. Nucleic acid isolation from rumen fluid from in vitro incubations Nucleic acids were isolated from 150 μl rumen fluid using a standard phenol-chloroform method and bead beating. DNA was obtained from nucleic acids using the Allprep DNA/RNA kit (Qiagen, Hildem, Germany) and quantified using Nanodrop (Thermo Fisher Scientific). qPCR of gene copies in rumen fluid Gene copies of total bacteria, RCC and non-RCC methanogens 16S rRNA genes, mcrA genes of all methanogens and the MA methyltransferase gene ( mttB ) genes of the RCC were determined by qPCR using primers summarized in Supplementary Table S6 . Primers for mttB were designed based on metatranscriptome reads. Cloning and sequencing of PCR amplicons confirmed their specificity. Primers 958 F and 1100AR were used to quantify 16S rRNA of non-RCC methanogens ( Methanobrevibacter, Methanomicrobium, Methanobacterium, Methanomicrococcus and Methanosphera ). These primers do not amplify RCC because of 1 and 3 bp mismatches [28] . qPCR was performed using a Mastercycler ep realplex (Eppendorf, Wien, Austria). Reaction mixtures (20 μl) contained 10 μl Qiagen QuantiFast SYBR Green PCR mix, 1 μl of each of the specific primers at a final concentration of 0.25 μM and 1 μl of template DNA. Running conditions were 95 °C for 5 min followed by 40 cycles of 95 °C for 10 s, 60 °C for 15 s and 72 °C for 30 s. Gene copies were calculated per μg DNA. For generation of plasmids to determine standard curves, the RCC 16S rRNA gene, mcrA and mttB, were amplified from rumen fluids, and PCR products cloned using pGemT-Easy Cloning (Promega, Fitchburg, WI, USA). For generation of standard curves of bacterial 16S rRNA and non-RCC methanogens, long fragments of PCR amplified 16S rRNA genes were used. Plasmids were linearized; plasmids and PCR products were diluted serially in 10-fold and applied as template in qPCR reactions. Melting curve analysis and agarose gel electrophoresis were performed to verify the identity of the genes of interest. Statistical analysis Data were statistically analysed using SigmaPlot (SigmaPlot 11; Systat Software) or Graph Pad. Effects of fat supplementation on SSU and mcrA gene transcripts of RCC and Methanobacteriales , as well as on bacterial and eukaryote SSU reads, were tested using paired t -tests. The impact of fat supplementation on CH 4 from CO 2 /H 2 , CH 4 from CH 3 -R and NH 4 + assimilation transcripts was evaluated using one-tailed paired t -tests. CH 4 in vitro production from TMA was tested using non-paired t -test. Gene abundances of methanogens and bacteria during in vitro fermentations were compared with one-way ANOVA applying the Holm-Sidak all-pairwise multiple comparison. Generally, P -values ≤0.05 and <0.001 were considered representing significant and highly significant effects of treatments, respectively, and P -values between >0.05 and ≤0.10 to represent trend-wise effects of treatments. Accession codes: Illumina raw sequence data is available through NCBI (Bioproject: PRJNA176598; Sequence Read Archive: SRA059441 ). How to cite this article: Poulsen M et al. Methylotrophic methanogenic Thermoplasmata implicated in reduced methane emissions from bovine rumen. Nat. Commun. 4:1428 doi: 10.1038/ncomms2432 (2013).